RETRACTED ARTICLE: Mechanically interlocked architecture aids an ultra-stiff and ultra-hard elastically bendable cocrystal Molecular crystals are not known to be as stiff as metals, composites and ceramics. Here we report an exceptional mechanical stiffness and high hardness in a known elastically bendable organic cocrystal [caffeine (CAF), 4-chloro-3-nitrobenzoic acid (CNB) and methanol (1:1:1)] which is comparable to certain low-density metals. Spatially resolved atomic level studies reveal that the mechanically interlocked weak hydrogen bond networks which are separated by dispersive interactions give rise to these mechanical properties. Upon bending, the crystals significantly conserve the overall energy by efficient redistribution of stress while perturbations in hydrogen bonds are compensated by strengthened π -stacking. Furthermore we report a remarkable stiffening and hardening in the elastically bent crystal. Hence, mechanically interlocked architectures provide an unexplored route to reach new mechanical limits and adaptability in organic crystals. This proof of concept inspires the design of light-weight, stiff crystalline organics with potential to rival certain inorganics, which currently seem inconceivable. Metals, metal-based alloys, and ceramics are typically stiff and hard due to their underlying strong metallic, covalent or electrostatic bonds, while molecular crystals with much weaker non-covalent interactions are softer [1] , [2] , [3] , [4] , [5] , [6] , [7] . For mechanical designs in materials engineering, light-weight along with high stiffness is highly desired. Despite molecular crystals being lighter and have shown enormous potential with several other advantages, such as in molecular electronics, non-linear optical applications, superconductors, and piezoelectrics [8] , [9] , [10] , [11] , [12] , [13] , [14] , [15] , their perceived softness and low load bearing ability prevented such considerations while the limits of their stiffness, hardness ( H, which is defined as the measure of resistance to plastic deformation), and toughness are yet to be fully established. Studies by Haussühl et al., using ultrasonic resonant frequency measurements on some hydrogen-bonded anisotropic molecular crystals showed exceptionally high E (elastic modulus, which is defined as a measure of resistance to elastic deformation) values for a few crystals in the range of 30 GPa to ~50 GPa, while β -succinic acid was the highest with ~120 GPa, corresponding to one of its crystallographic directions [16] , [17] . So far, such high stiffness is thought to occur only in crystals with strong hydrogen bond networks, e.g., by N–H···O, O–H···N, O–H···O, etc [18] , [19] , [20] . Moreover, it is perceived that the exceptionally stiff and hard crystals are brittle and not flexible. On the other hand, mechanical elastic flexibility is seen only in certain softer single crystals (<20 GPa) with predominantly weaker (dispersive) interactions [3] , [4] , [21] , [22] . This seems that high stiffness and elastic flexibility is mutually exclusive and combining the two is a challenge. Recent studies on mechanism of elastic bending of molecular crystals using in situ three point bending and Raman spectroscopy showed an evidence of heterogeneous molecular changes in the structure [23] . Worthy et al., using micro X-ray diffraction, demonstrated in a coordination compound, Cu(acac) 2 , that mutual rotation of molecules facilitate expansion at the outer arc and compression at the inner arc within its 1% elastic limit while extending the argument to plastic nature at higher strains [21] . However, it is not known whether such mechanisms from simple non-hydrogen bonded systems extend to other elastic crystals with hydrogen bonding and mechanical interlocking in the structure. Furthermore, the fate of mechanical properties and energetics, post bending and reversibility of elastic crystals is yet to be established. On the other hand, naturally born complex architectures in bones, teeth, seashells, collagen and spider silk that aid remarkable combination of properties, such as stiffness, strength, flexibility, healing, or hardness, have sparked tremendous interest among scientists to investigate bioinspired structural materials [24] , [25] , [26] , [27] , [28] , [29] . Rational design of composite crystals via occlusion of few molar proportions of aspartic acid and glycine amino acids have demonstrated exceptional hardening of calcite crystals from 2.5 GPa to 4.1 GPa [30] . However cocrystals, which have been exploited to alter the physicochemical properties of pharmaceuticals [31] , ferroelectrics [32] , optoelectronics, and charge transfer materials [33] , have not been perceived as composite materials. Unlike conventional composites, which typically have at least two sub-lattices, cocrystals have a single lattice with homogenous distribution of constituent molecules [34] . The heterogeneity in cocrystals can be introduced at structural level by carefully exploiting directional and dispersive intermolecular interactions, to access properties that are remarkably different from individual coformers. The elastic bending nature of the cocrystal solvate of caffeine (CAF), 4-chloro-3-nitrobenzoic acid (CNB) and methanol (1:1:1) was reported by us earlier [35] , [36] , but quantification of its mechanical properties and bending mechanism remained intriguing, when compared to other elastically bendable molecular crystals known today [2] , [10] , [21] , [22] , [23] , [37] , [38] , [39] , [40] , because this is the only system with weak hydrogen bonded, mechanically interlocked network. Hence, we reinvestigated its elastic bending using spatially resolved analysis up to atomic resolution by employing state-of-the art single crystal micro ( μ ) X-ray diffraction ( μ -SCXRD), μ -Raman and μ -Infrared ( μ -IR) spectroscopy, on both as grown (or ambient) and bent crystals. The complete structural analysis including energy frameworks calculations reveals that the mechanical interlocking aids not only elastic flexibility in this cocrystal, but also the exceptionally high stiffness [41] and hardness. Notably, these mechanical properties are very distinct from that of the individual components. Quantification of exceptional elastic modulus and hardness Quantitative nanoindentation experiments were performed on the (010) major and (001) minor faces (Fig. 1a ; Supplementary Figs. 1 – 5 ) of ambient single crystals using a Berkovich indenter tip. P–h characteristics at both the faces exhibit significant recovery showing their elastic nature and resistance towards permanent deformation (Fig. 1b ). The loading curves are smooth without pop-ins discarding possibilities of sudden slippage of molecular layers [6] . Curves for the major (010) face are smoother with a lower penetration depth as compared to the minor (001) face. 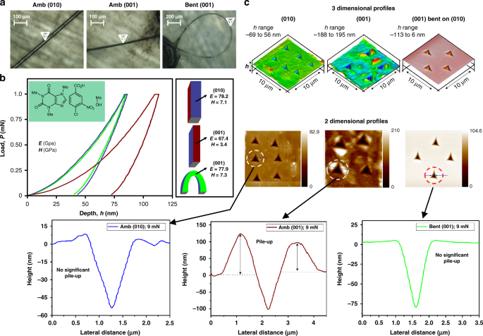Fig. 1 Mechanical properties of ambient and bent crystals obtained by nanoindentation.aOptical images of (010) and (001) of straight crystals and (001) face of the crystal loop bent on (010) and schematic indenter tip (white cone).bLoad–depth (P–h) curves obtained on an ambient cocrystal from indentation on (010) (blue), (001) (brown) face and a bent crystal, on (001) (light green) face and their corresponding highestEandHvalues.cIn situscanning probe 3D and 2D microscopic images of impressions at 9 mN load with corresponding height profiles of impressions elucidating pile-up characteristics of different faces of ambient and bent crystals Measured elastic modulus ( E ) for (010) was found to be as high as 76.86 (±1.30) GPa while for (001) face was 64.39 (±1.96) GPa (Table 1 ). These exceptionally high values are comparable to certain metals, such as aluminum, which has density nearly double to that of the cocrystal (1.48 gcm −3 ). These E values are almost nine-fold and five-fold larger than that obtained on single crystals of pure CAF (8.73 GPa) [42] and CNB (14–16 GPa), respectively (Supplementary Table 1 and Supplementary Fig. 6 ). H of the cocrystal was also found to be exceedingly high, 6.92 (±0.19) GPa for (010) and 3.23 (±0.13) GPa for (001) (Table 1 ). The H values of (010) are also highest among molecular crystals (typical range of H is ~0.1–1.5 GPa; highest known from nanoindentation is ascorbic acid, ~5.6 GPa) [43] , [44] . These H values are of the range of glasses (5–10 GPa) and larger than that of commercially available stainless steel (~5 GPa) [45] . The results therefore counter the general perception of relating all organic crystals to softness, particularly, the flexible ones. Fig. 1 Mechanical properties of ambient and bent crystals obtained by nanoindentation. a Optical images of (010) and (001) of straight crystals and (001) face of the crystal loop bent on (010) and schematic indenter tip (white cone). b Load–depth ( P – h ) curves obtained on an ambient cocrystal from indentation on (010) (blue), (001) (brown) face and a bent crystal, on (001) (light green) face and their corresponding highest E and H values. c In situscanning probe 3D and 2D microscopic images of impressions at 9 mN load with corresponding height profiles of impressions elucidating pile-up characteristics of different faces of ambient and bent crystals Full size image Table 1 Elastic modulus ( E ) and hardness ( H ) obtained on ambient (010) and (001), and bent (001) faces of single crystals of the cocrystal at different indentation loads Full size table E and H values, post mechanical bending, were also investigated by bending the cocrystal on (010) major face into a loop while indenting perpendicular to the (001) face at the acutely bent region. The E value has significantly increased by ~12% [76.12 (±1.42) GPa] while the H increases two-fold [7.30 (±0.02) GPa] (Table 1 ). The increased stiffness and hardness upon mechanical perturbation bear evidence to stiffening and hardening upon mechanical bending. Structural basis for exceptional mechanical properties Crystal structure obtained using synchrotron μ -SCXRD at ambient temperature [orthorhombic space group Fdd 2, V amb = 7664(2) Å 3 ] is consistent with the reported form [35] (Refcode: BEDYIU; Supplementary Tables 2 – 6 ; Supplementary Fig. 7 ). In the structure, the CAF and CNB molecules form dimers via strong O–H···N ( d /Å; θ /°: 1.56 Å, 177°) and C–H···O (2.65 Å, 120.72°) hydrogen bonds (Fig. 2a ). The CAF molecules of adjacent dimers are connected via weak C–H···O (2.55 Å, 140.65°) bonds forming one dimensional (1D) extended chains running along two cross directions [103] and [10-3], which are oriented at an angle of 40.98° with respect to each other (Figs. 2a, b ). The CNB molecules of alternate dimers fall on either side of the 1D chains making them double-sided comb-like tapes (Fig. 2a ). The peripheral CNB molecules (teeth) from adjacent tapes close pack via dispersive interactions, leading to mechanical interlocking, practically making the arrangement like a zipper. The tapes further pack along c -axis via π -stacking interactions between CAF–CAF and CNB–CNB pairs (Fig. 2b ). The solvent methanol molecules form channels parallel to c . Note that only the CAF–CNB dimers (0D) involve strong O–H···N hydrogen bonds, while the 1D chains (CAF–CAF) are primarily supported by the weak C–H···O. Hence the zipper network is primarily based on weak interactions. Fig. 2 Crystal packing and schematic representation of resistance to external load. Geometry and packing of the comb-like tapes (blue-green shades) viewed along c ( a ) and along b ( b ). The zipper-like conformation of the comb-like tapes resists deformation by knuckling, sliding and compression against external load on (010) and (001) faces. Inset of a shows the atom labels with intermolecular interactions. Molecular graphics with thermal ellipsoids can be found in Supplementary Fig. 8 Full size image Notably, the tapes in the center are populated with polar groups while the exterior is dominated mainly by van der Waals groups (Fig. 2a ). The packing of the cocrystal is unique due to several levels of mechanical interlocking. The zipper type locking resists movement of molecules along the direction of the tapes as well as in the orthogonal directions to their length under external mechanical stress. Upon application of load on major face (010), interlocked comb-like tapes exert strong resistance to knuckling along b and sliding along a (compare Figs. 2a, b ), resisting any plastic slippage. These structural features may be responsible for the large E and H values obtained on the (010) face. On the other hand, upon indentation on the minor face (001), i.e., parallel to c -axis, the π -stacking interactions provide the room for compression or sliding of molecules locally, while the interlocking resists rupture (Fig. 2 ), which is why the E and H values are lower compared to that of (010), but large compared to typical molecular crystals. The significant pile-up of material observed on the (001) face after unloading reveals the incompressible plastic deformation nature of this face (Fig. 1c , Supplementary Figs. 3 and 4 ). As the crossed 1D tapes make a slope with respect to the (001) face (Fig. 2b ), the molecules slide in the direction of these tapes and the material extrudes on the top surface when sufficient indentation force is applied [46] . Spatially resolved structural changes in bent crystal We have investigated the associated atomic-level structural changes by carrying out μ -SCXRD using synchrotron radiation with a beam size of 1.63 (vertical) × 3.50 (horizontal) μm 2 . We could achieve the data completeness of 56% up to resolution of (sin θ/λ) max ≈ 0.65 Å −1 ( F -centered point group symmetry mmm ), which enabled us to individually perform structure solutions and refine the crystal structures (see Supplementary Notes 1.1 and 1.2 ; Supplementary Table 4 ). The μ -IR and μ -Raman spectroscopy experiments have been performed to independently validate these results and study the changes in the vibrational modes of –CH groups taking part in intermolecular C–H····O bonds and π -stacking, because standard structure refinements are limited to riding model for the hydrogen atom positions. 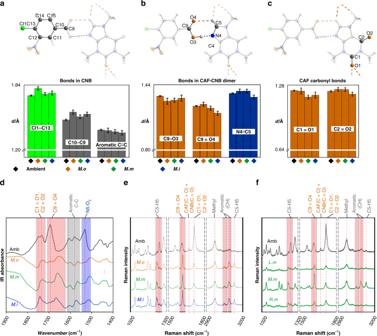Fig. 4 Analysis of bond modulations using X-ray and spectroscopy data.a,b,cHistogram plots showing changes in some important covalent bonds in CNB (a), CAF–CNB dimer (b), and carbonyl groups of CAF (c) in crystal structures atM.o,M.m, andM.i.dμ-IReunpolarized Raman spectra on ambient (grey square) and the bent crystal at midpoint (orange =M.o, green =M.m, blue =M.i);fComparison ofμ-Raman spectra ofM.m,L.m,R.mand ambient. Width of the coloured blocks within the IR and Raman spectra represents the magnitude of shifts of corresponding covalent bands. Absolute errors are given ina,b,c. Calculated IR and Raman spectra in Supplementary Fig.9and Supplementary Table6 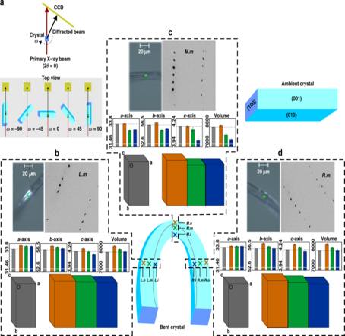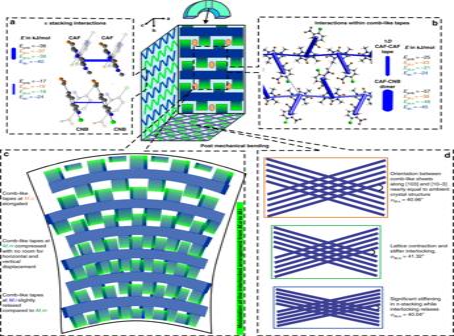Fig. 5 Schematic description of structural changes. Total interaction energiesarelated toπ-stacking between pairs of CAF–CAF and CNB–CNB, andbamong molecules within comb-like 1D tapes in ambient and regions ofM.cSchematic representation of the strained interlocked tapes depicting elongation, compression and slight relaxation at regions ofMof bent crystal viewed along [001] direction.dChanges in stacking and the angle among tapes. Solvent molecules are omitted for clarity The spatially resolved μ -SCXRD, performed at the midpoint, M , right, R , and left, L , shoulders of the bent crystal loop, revealed several interesting factors related to elastic bending mechanism (Figs. Fig. 3 Spatially resolvedμ-SCXRD analysis of mechanically bent crystal.aSchematic representation of the strategy employed inμ-X-ray diffraction data collection. Inb,c, andddiffraction peaks, optical images of region of crystal loop, histogram plots of distribution of lattice parameters and boxes representative of schematic unit cells (dark gray =ambient, orange =outer, green =middleand blue =inner) at thebleft shoulder (L),cmidpoint (M), anddright shoulders (R). The schematic boxes are drawn while multiplying five times the percentage changes. The neutral axis (an axis in the cross section of the beam along which structural perturbations are minimal) of the bent crystal is outward atMand inward atLandR, and not at the midpoint of the cross section35. Absolute error bars are provided in the histogram plots 3 , 4 , and 5 ) that are radically different from the plastic crystals [6] and earlier models of elastic crystals [2] , [21] , [22] , [40] . At each of these three locations, M , R , and L , we collected the data at outer ( o ), middle ( m ), and inner ( i ) cross sections of the arc and obtained sharp Bragg reflections with comparable profiles. This confirmed the presence of long range order probed within the spatial resolution of our technique (Figs. 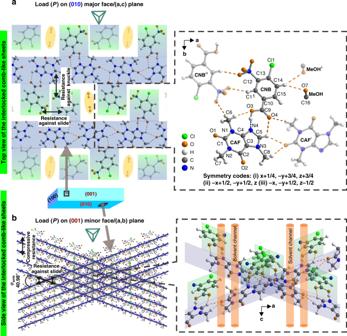3b, c, d ; Supplementary Fig. 7 ). With respect to the volume of ambient crystal ( V amb = 7664 Å 3 ), the average volume at M showed a contraction (-3.29%), but surprisingly a slight expansion was observed at L (1.55%) and R (1.60%). Fig. 2 Crystal packing and schematic representation of resistance to external load. Geometry and packing of the comb-like tapes (blue-green shades) viewed alongc(a) and alongb(b). The zipper-like conformation of the comb-like tapes resists deformation by knuckling, sliding and compression against external load on (010) and (001) faces. Inset ofashows the atom labels with intermolecular interactions. Molecular graphics with thermal ellipsoids can be found in Supplementary Fig.8 This long range redistribution of stress allows the crystal to conserve the volume (average of V M , V L , and V R of the bent crystal is = 7598.5 Å 3 ; Supplementary Table 2 ). The effect of perturbation on structure along cross sections is highly anisotropic. The magnitude of compression from the outer to the inner arc at the M (−7.34 %) is extraordinarily high, and it is moderate at the shoulders ( L = −2.68 % and R = −3.15 %). This anisotropic shrinkage is primarily due to the large changes in c -axis (−4.05% for M ; −1.67 % for L ; −1.92% for R ) (Figs. 3b–d ; Supplementary Table 2 ), revealing the adaptability of this axis. Along this direction, π -stacking and methanol solvent channels are present. Note that the c -axis is perpendicular to the applied bending force. This suggests that the compression is dependent on the nature of the crystal and not solely on the direction of the applied force. The increased E and H are possibly a result of enhanced π -stacking interactions. The a and b axes also show significant contraction from M.o to M.m (−1.85% and −2.13%, respectively) while slight relaxation from M.m to M.i (0.21% and 0.42%, respectively), exhibiting modulation rather than monotonous decrease. The plateauing trend of the a and b axes depicts the crystal’s resistance to further contraction. Fig. 3 Spatially resolved μ -SCXRD analysis of mechanically bent crystal. a Schematic representation of the strategy employed in μ -X-ray diffraction data collection. In b , c , and d diffraction peaks, optical images of region of crystal loop, histogram plots of distribution of lattice parameters and boxes representative of schematic unit cells (dark gray = ambient , orange = outer , green = middle and blue = inner ) at the b left shoulder ( L ), c midpoint ( M ), and d right shoulders ( R ). The schematic boxes are drawn while multiplying five times the percentage changes. The neutral axis (an axis in the cross section of the beam along which structural perturbations are minimal) of the bent crystal is outward at M and inward at L and R , and not at the midpoint of the cross section [35] . Absolute error bars are provided in the histogram plots Full size image Fig. 4 Analysis of bond modulations using X-ray and spectroscopy data. a , b, c Histogram plots showing changes in some important covalent bonds in CNB ( a ), CAF–CNB dimer ( b ), and carbonyl groups of CAF ( c ) in crystal structures at M.o , M.m , and M.i . d μ -IR e unpolarized Raman spectra on ambient (grey square) and the bent crystal at midpoint (orange = M.o , green = M.m , blue = M.i ); f Comparison of μ -Raman spectra of M.m , L.m , R.m and ambient. Width of the coloured blocks within the IR and Raman spectra represents the magnitude of shifts of corresponding covalent bands. Absolute errors are given in a , b, c . Calculated IR and Raman spectra in Supplementary Fig. 9 and Supplementary Table 6 Full size image Fig. 5 Schematic description of structural changes. Total interaction energies a related to π -stacking between pairs of CAF–CAF and CNB–CNB, and b among molecules within comb-like 1D tapes in ambient and regions of M . c Schematic representation of the strained interlocked tapes depicting elongation, compression and slight relaxation at regions of M of bent crystal viewed along [001] direction. d Changes in stacking and the angle among tapes. Solvent molecules are omitted for clarity Full size image To provide a complete crystal chemical analysis of strained regions, M.o , M.m , and M.i, we refined the structures with atomic displacement parameters (ADPs) using both isotropic and anisotropic description, for all non-hydrogen atoms, but the refinements for the former yielded poor fit to the diffraction data and chemically non-meaningful distances, hence only the anisotropic descriptions are considered for further structural analysis (see Supplementary Note 2.2 , Supplementary Tables 3 and 5 ). The strained regions, M.o , M.m , and M.i revealed anisotropic changes in intermolecular interactions (Fig. 4 ). The most adversely affected site is the hydrogen bonded CNB–CAF dimer (Fig. 4b ). For instance, the (CNB) C = O bond shortens from M.o to M.i [ d C=O = 1.25(2) to 1.16(2) Å] and the (CNB) C–O bond is nearly same ( d C–O = 1.28(3) to 1.31(3) Å). We have also noticed similar anisotropy (change/no change) in the nitrogen to carbon distances in the five-membered ring of CAF [ d N4–C5 = 1.38(2) to 1.32(2) Å, d N4–C4 = 1.36(2) to 1.34(2) Å]. The other peripheral bonds change to a lesser extent [eg. d C–Cl = 1.80(2) to 1.75(2) Å] while the inner ring bonds are marginally affected [aromatic d C–C = 1.40(3) to 1.36(3) Å] [compare Fig. 4 (b) to (a) and (c)]. Orientation between mean planes of CAF and CNB molecules in this dimer ( M.o = 6.11°; M.m = 5.6°; M.i = 5.93°) also changes with respect to the ambient structure (4.98°). The C1 = O1 group of CAF molecule that forms 1D tapes, contracts from M.o to M.m and then slightly elongates towards M.i (Fig. 4c ). The observed changes reveal the high modularity of the structure. The changes in the bonds of CAF–CNB dimer are in line with their resistance against slip (due to mechanical interlocking) under external bending stress. In the μ -IR spectra, the (CNB) ν (C9 = O4) shows the largest blue shift from M.o to M.i region suggesting the weakening of interactions of the CNB–CAF dimer (Figs. 4b, d , Supplementary Fig. 9b ). The carbonyl groups of CAF, which involve in forming 1D chains also show blue shift in IR, but to a lesser extent. This is consistent with the observed large changes in bond distances in CAF–CNB dimer (teeth of the tape) than in CAF–CAF (central part of the tape) interactions in crystal structures [compare Fig. 4 (d) to (a) and (b)], hence gives credence to the trends observed in the μ -SCXRD analysis. Most bands recorded at M are red-shifted with respect to ones at ambient, which reflects weakening of these covalent bonds due to overall lattice perturbations arising from anisotropic mechanical stress. In the unpolarized Raman spectrum measured at the position M of the crystal loop, the 1612 cm −1 band at ambient for (CNB) ν (C9 = O4) blue shifts to 1617 cm −1 in all regions from outer to inner (Fig. 4e ), which suggests that this bond gets stiffer, while the symmetric stretching band (CAF) ν (C5-H5) at 3085 cm −1 is significantly stronger at all regions of M as compared to ambient inferring its decreased polarizability and weakening of C–H···O interactions both within the dimer and CAF–CAF. However, the in plane bending mode of (CAF) ν (C5–H5) is red-shifted (1259 cm −1 at ambient, 1238 cm −1 at M ) (Figs. 4b, d ). This is a possible indication of strengthened π -stacking interactions amongst CAF molecules. Different degrees of strain exerted on different locations of the comb-like tapes [compare Figs. 4 (a), (b), (c)] leads to the suppression of the synchronized vibrations of (CNB) C = O and (CAF) C = O observed at 1672 cm −1 in the ambient crystal. On the other hand, symmetric stretching bands corresponding to aromatic C–H groups of the CNB at 3089 and 3065 cm −1 show red shift supporting considerable strengthening of π -stacking interactions along c at all the regions of M (consistent with shrinkage of c -axis as shown in Fig. 3 ). In the Raman spectra at the shoulders, bands corresponding to the (CAF) C = O, synchronized (CAF+CNB) C = O and C–H at higher wavenumbers largely resemble that of the ambient one while the (CNB) C = O is blue-shifted (Fig. 4f ), showing traits intermediate to the ambient and M regions. Energetic basis of elastic bending and higher stiffness We have determined pairwise total intermolecular interaction energies ( E total ) from energy frameworks calculations on the four experimentally determined structures (amb, M.o , M.m , and M.i ) using CrystalExplorer17 [47] , [48] , [49] software and confirmed that (i) the dominant feature of the structure is stacked comb-like tapes, (ii) the increased E and H values are a result of enhanced π -stacking interactions, and (iii) stress distribution is anisotropic along different directions at different regions of the bent crystal (Figs. 5a, b ; Supplementary Fig. 10 , Supplementary Tables 8 and 9 ). The comparison of E total of the dimer, CAF–CNB, of ambient crystal (−57 KJmol −1 ) with that of the M.o , M.m , and M.i (−38, −48, and −45 KJmol −1 ) reveals the decrease in overall stability in the stressed crystal. The CAF–CAF interactions in ambient (−25 KJmol −1 ), and M.o , M.m , and M.i (−23, −21, and –24 KJmol −1 , respectively) also show overall weakening of intra-tape interactions, but are less pronounced, and are in excellent agreement with the μ -SCXRD and μ -Raman results. On the other hand, the E total for π -stacking interactions among CNB–CNB and CAF–CAF pairs showed an opposite trend and become stronger at the strained regions, M.o (−19 and −37 KJmol −1 ), M.m (−18 and −40 KJmol −1 ), and M.i (−24 and −40 KJmol −1 , respectively) as compared to the ambient (−17.3 and −36.0 KJmol −1 , respectively). Comparison of aggregate E total of all molecules involved in hydrogen bonds, in ambient structure (−93 KJmol −1 ) and the strained structures at < M > (−75 KJmol −1 ), reveal ~19% loss in stability. On the contrary, ~11% strengthening is observed in the π -stacking interactions at M . This suggests that stability lost by the strained hydrogen bonds is compensated by the π -stacking interactions, making the total loss only ~8%. Note that stronger π -stacking interactions and stiffened interlocking of tapes further resist the deformation, thus leading to increase in E and H in nanoindentation on the (001) face of the bent crystal. The detailed spatially resolved data and energy frameworks analyses suggest that the mechanical interlocking of comb-like tapes play a major role in the exceptional mechanical properties while the modular nature of the structure aids elastic flexibility in these crystals. Upon bending, the mechanically interlocked structure efficiently redistributes the stress on a large number of molecules in a reversible manner rather than assisting plastic deformation. Contrary to the earlier proposed monotonous structural contraction of unit cell parameters [21] from outer to inner arc in elastically bendable crystals, here we observed a plateauing behavior towards the crystal’s boundary of the inner arc. This suggests to a complex mechanism with synergistic effects between directional and non-directional interactions leading to significant energy and volume conservation (Fig. 5 ). The external mechanical stress perturbs the intermolecular interactions, covalent bonds, as well as mutual orientation of the tapes (Figs. 5c, d ). Generally, a thermodynamically stable crystal is a result of trade-off among various types of intermolecular interactions where the stronger interactions typically play a dominant role while the weaker ones are compromised. Here the bending of crystal causes anisotropic strain in the mechanically interlocked tapes, leading to weakening of hydrogen bonding interactions. This reduces the dominance of directional interactions, making it conducive for the π -stacking to strengthen. The resistance to plastic deformation and storage of large amount of elastic strain in the distorted bonds, all point towards the system’s tendency to revert back to its pristine state. Here we showed an extraordinary mechanical stiffness and hardness in an elastically bendable crystal, in which the stress is distributed and stored over a large number of molecules (at crystal level), leading to short range reversible perturbations at molecular length scale. Contrary to the mechanical softening observed (lowering of H and E ) [6] in plastically bendable crystals (due to defects), here we showed hardening and stiffening in the elastic crystals. This could be a general phenomenon in elastic crystals, but the magnitude of hardening and stiffening will depend on the structural changes and resistance to plastic deformation. The present extensive methodical analysis also answers some unresolved problems and counters common perceptions regarding elastically bendable crystals; (1) Molecules in elastically bent crystals are not only related by rotation along the arc but also could show significant differences in their internal geometry and intermolecular interactions, as confirmed by μ -SCXRD and μ -Raman studies; (2) The neutral axis not necessarily lies at the mid-plane of the crystal, but may shift towards the expansive arc at the middle and towards the compressive side at shoulders of the loop; and (3) The overall volume of the crystal is conserved in bent state (overall contraction at M region and expansion at shoulders, L and R ). Worthy et al. suggested that the mechanical interlocking is not necessary for elastic flexibility in organic crystals [21] , [50] . This should be seen in the following context. Every crystal can bend elastically, including crystals of diamond [51] . Particularly, the molecular crystals, which have relatively weaker bonds (compared to inorganic counterparts), can typically take strains of ~0.5–1% and much beyond. The elastic deflection in acicular morphologies (wires) is easier to notice at macroscopic scale but the extent of elasticity (% of strain) is determined by the material’s internal structure and its ability to prevent plastic flow and fracture. Crystal packing without mechanical interlocking and with weak interaction planes (as in the case of Worthy et al.) [21] may allow some initial elastic flexibility (due to energetic barriers or elastic energy), but the absence of mechanical resistance to slip may eventually assist plastic deformation (irreversible) [21] , hence only limited elasticity is expected. When such anisotropic crystals with weak interaction planes break under excess mechanical stress, the pieces may not recover from the bent shape completely (elasto-plastic nature) [52] . However, crystals with mechanically interlocked weak interaction planes and superior elastic nature (with strains over ~2-3%) may recover fully. It is important therefore to distinguish between elasto-plastic, plastic and highly elastic crystals based on the magnitude of strain they can withstand and associated structural features (e.g,. mechanical interlocking, rugosity, or topology of the slip plane). The significant atomic-level anisotropic changes in functional elastic crystals may facilitate tuning physical properties through external mechanical stimuli. Mechanically interlocked architectures in covalent systems have been of great interest in supramolecular chemistry and molecular motors [53] , and here we showed their significance in the context of molecular crystals. It would be important to explore other mechanically interlocked topological structures and supramolecular interactions for going beyond the perceived limits of molecular crystals and to design attractive adaptive solids for materials engineering and biomimetics [54] , [55] , [56] , [57] . Material synthesis Long single crystals of dimension ~10 × 0.03 × 0.02 mm 3 of the cocrystal solvate were obtained by mixing equal molar solutions of CAF and CNB in methanol employing slow evaporation method. The (010) face is the major face (~10 × 0.03 mm 2 ) while (001) face is the minor one (~10 × 0.02 mm 2 ) 1 . Nanoindentation For ambient (straight as synthesized) cocrystal, single crystals were carefully mounted on the coverslip using minimal amount of super glue (Fevi kwik) and the coverslip was then further glued on top of a steel stub, in such a way to avoid any issues in machine compliance. Another batch of single crystals were bent (on 010 face) into a loop (as shown in Supplementary Fig. 2d ) and then fixed on the coverslip by using super glue, following the same procedure used for the ambient crystals. Nanoindentation experiments have been done using the instrumentation set up from Hysitron Triboindentor, TI Premier, Minneapolis, USA equipped with an in situ Scanning Probe Microscope (SPM) employing a Berkovich tip having an effective radius of 150 nm. Area function calibration has been done by doing indentation on fused quartz as standard sample and was fit to the data using a classic Hertzian loading profile [58] . Single crystals of both as synthesized and bent were probed up to load of 1, 4, and 9 mN with loading/unloading rate of 0.2, 0.8, and 1.8 mN/s, respectively, with a hold interval of 2 s before unloading. Hardness and elastic modulus have been determined using the standard Olive-Pharr (O&P) method [58] , [59] . The single crystals of the cocrystal were generally very thin compared to other organic samples probed using nanoindentation in literature. Initially, several single crystals were probed for measuring E and H values. Some crystals yielded lower E and H values with large standard deviations and with poor indentation impression. This is attributed to poor crystal quality, surface roughness and machine compliance issues [60] . The crystals, which yielded highest E and H values, were of highest quality and also gave very consistent data and excellent impressions with small standard deviations. These results were reproducible from single crystals obtained from different batches, which are presented in the article. Micro-X-ray diffraction Single crystals in ambient and bent shape were fixed separately on a nylon loop using silicon grease for diffraction experiments. X-ray diffraction measurements with a micro-X-ray beam were carried out using the precision diffractometer in the SPring-8 BL40XU beamline. The X-ray beam ( λ = 0.78210 Å) was focused to 1.63 (vertical) × 3.50 (horizontal) μm 2 using a zoneplate. To irradiate only a focused beam, a 30-μm diameter order sorting aperture (OSA) and a 40-μm-diameter centerstop were used. The focused X-ray was incident normal to the bending plane ( ω = 0°). The ω range, oscillation angle (Δ ω ) and exposure time were ±90°, 3° and 3 s for bent crystal loop and ±90°, 2° and 2 s for ambient crystal, respectively. The measurements were performed at room temperature and diffraction images were measured with a Rigaku Saturn 724 charge-coupled device (CCD) detector. For the data collections at inside and outside position of the bent single crystal, the measurement positions were 5 μm inside and outside from the middle of the crystal, and 60 diffraction images were collected from each position. 90 diffraction images were collected for the ambient crystal. Data reductions have been performed using the software suite CrysallisPro [61] . Structure solutions and refinements have been performed using SHELXT [62] and JANA 2006 [63] , [64] , respectively. Micro-Infrared spectroscopy For micro-Infrared spectroscopy measurements, the bent crystals were glued on a sample stage using silicone grease. Measurements were performed at beamline BL43IR, SPring-8 with a Vertex70 FTIR spectrometer, and a Hyperion2000 infrared microscope from Bruker. Spectra have been recorded from 600 to 4000 cm −1 with 2 cm −1 resolution and accumulation of 256 and 64-fold with normal infrared. The infrared beam was focused to 10 (vertical) × 10 (horizontal) μ m 2 with a knife-edge aperture in the microscope. Micro-Raman spectroscopy For micro-Raman spectroscopy single crystals were made into loop by bending while gluing both the ends on a coverslip. Spectra were recorded on ambient and bent crystals in the range 100–4000 cm −1 with a micro-Raman spectrometer LABRAM HR from Horiba Jobin Yvon with a 1800 groves per mm grating. Laser spot on the samples was focused to ~1 μ m using a 100x zoom lens. All measurements were performed employing wavelength of 632 nm (He–Ne laser) at 10 s exposure time. DFT computational details All calculations were performed by implementing the Gaussian 09 [65] Quantum Mechanics package. The molecular structures obtained from the .cif file of the ambient crystal were converted to .pdb format. The structures were then optimized and their respective frequency calculations were conducted using the Density Functional Theory (DFT) with a B3LYP-D2/631G**(d,p) basis set, which has shown effectiveness in Raman and IR vibrational mode calculations. Obtained spectra were then compared to experimentally observed results on the systems of interest and were found to be in good accordance, after which the vibrational modes observed in experiment were assigned by correlating the wavenumbers of the calculated modes (Supplementary Fig. 9 , Supplementary Table 6 ). Energy frameworks calculations Energy frameworks calculations pertaining to intermolecular interactions were performed using the software suite CrystalExplorer 17 [47] , [48] , [49] , [66] , [67] based on Gaussian B3LYP-D2/6-31G(d,p) molecular wave-functions calculated using .cif files obtained from the ambient crystal and M.o , M.m , and M.i regions of the bent crystal loop using experimental crystal geometries, with X–H bond lengths normalized to standard neutron diffraction values. Pairwise interaction energies between molecules were calculated considering radius of 3.8 Å from centroid of a molecule to an atom (of another molecule) belonging to its nearest neighbor. The present system is a multi-component crystal. Hence, energies were calculated separately by choosing each molecule in the asymmetric unit, one at a time. Calculations based on disordered conformation of the nitro group yielded physically non-meaningful energies, which is why an ordered approximation was imposed. The energy framework was constructed based on the crystal symmetry and total intermolecular interaction energy (E_tot), which includes electrostatic (E_ele), polarization (E_pol), dispersion (E_dis), and exchange-repulsion components (E_rep) with scale factors of 1.057, 0.740, 0.871, and 0.618, respectively. Where E_total = 1.057E_ele + 0.740E_pol + 0.871E_disp + 0.618 E_rep. (Supplementary Fig. 10 , Supplementary Tables 7 and 8 ).